Gene network reconstruction reveals cell cycle and antiviral genes as major drivers of cervical cancer Although human papillomavirus was identified as an aetiological factor in cervical cancer, the key human gene drivers of this disease remain unknown. Here we apply an unbiased approach integrating gene expression and chromosomal aberration data. In an independent group of patients, we reconstruct and validate a gene regulatory meta-network, and identify cell cycle and antiviral genes that constitute two major subnetworks upregulated in tumour samples. These genes are located within the same regions as chromosomal amplifications, most frequently on 3q. We propose a model in which selected chromosomal gains drive activation of antiviral genes contributing to episomal virus elimination, which synergizes with cell cycle dysregulation. These findings may help to explain the paradox of episomal human papillomavirus decline in women with invasive cancer who were previously unable to clear the virus. Although it has been known for decades that persistent infection with high-risk human papillomavirus (HPV) is the major risk factor for the development of cervical cancer [1] , the exact means by which the virus induces tumour growth and the genomic changes that promote tumours have not been completely elucidated [2] . On the one hand, it is known that failure to mount an effective immune response facilitates viral persistence and integration into a host genome leading to genomic aberrations and a subsequent development of cervical cancer after several decades [3] . Episomal virus can cause some genomic instability during early stages of viral infection even before integration into a host genome [4] , [5] . On the other hand, there is evidence that the loss of episomal HPV is important in disease progression after virus integration. For example, data from biopsies suggest that precancerous lesions have more episomal virus than high-grade tumours [6] , [7] , and data from cervical cell lines show that cervical keratinocytes that lose episomal virus show increased expression of viral oncogenes coded by the integrated form [8] . This increase seems to be due to the loss of the regulatory viral gene, E2 , which is frequently disrupted on integration, and which normally suppresses the expression of the viral oncogenes E6 and E7 ( [2] ). The E6 and E7 transforming proteins have multiple mechanisms to alter cell cycle control and to cause genomic instability that lead to an increase of chromosomal aberrations and mutations in cellular genes [9] . The loss of episomal virus in the in vitro cell lines coincides with an increase of antiviral immune response, and this has led to another model of carcinogenesis, suggesting that an augment in antiviral activity results in the elimination of episomal virus aiding tumour progression [8] . There are thus two main questions that are currently awaiting answers: is there evidence of a similar antiviral immune response in cervical tumours in vivo and, if yes, why would women that have not been able to deal with HPV infection for a long time suddenly acquire an antiviral response strong enough to generate a dramatic decrease of viral load? Here we sought to identify in unbiased way molecular mechanisms and key gene drivers that may be involved in the cervical carcinogenesis using an integrative systems biology approach. Although we did not originally aim to ask the above questions, our results have positively answered the first question and provided the basis for solution of the paradox contained in the second one. We started by generating gene expression data from 40 tumours and 20 normal tissue samples. Combining these data with data from four other independent studies, we revealed a robust set of differentially expressed genes (DEGs) and used it to reconstruct a gene coexpression network of cervical cancer. We found three major subnetworks, one containing genes involved in the cell cycle, another related to the antiviral activity, and a third minor network related to epithelial cell differentiation. Integrating these data with data on genomic (chromosomal) aberrations, we found that the cell cycle and antiviral subnetworks were regulated by genes located within the same regions of chromosomal amplification. We suggest that the activation of antiviral genes that occurs late in women that have not otherwise made strong this response is driven by selected chromosomal changes in HPV-transformed cells. We propose a model in which frequent aberrations contain regulatory genes that stimulate the antiviral response and the cell cycle, and consequently promote the elimination of inhibitory episomal virus and uncontrolled proliferation, allowing the dysplastic cell to become a malignant tumour. Chromosomal aberrations regulating gene expression We performed a meta-analysis of gene expression microarray data using our data set and four others from the literature ( Supplementary Table S1 ) to identify genes with altered expression in cervical tumour samples versus normal tissue. We identified 1,268 genes with a false discovery rate (FDR) <1%, of which 526 genes were downregulated in tumour samples (Down-genes) and 742 genes were upregulated (Up-genes) ( Fig. 1a , Supplementary Data 1 ). 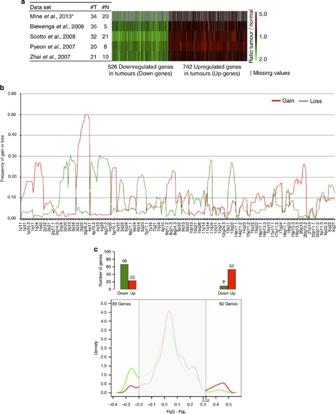Figure 1: Chromosomal aberrations regulating expression of genes from frequent chromosomal gain or loss. (a) Heat map of the 1,268 genes differentially expressed between cervical tumour and normal tissue samples in the five data sets used for the meta-analysis of gene expression microarray data. red-upregulated, green-downregulated, grey-missing value. *Current study. (b) FqG (red) or loss (FqL, green) in the genome detected in the meta-analysis of comparative genomic hybridization studies using cervical cancer samples. (c) Distribution of the delta values (FqG—FqL) for the 1,268 genes. Chromosomal regions with delta values >0.32 or <−0.2 were considered to be the regions of frequent gains or losses, respectively. Bar graph shows the number of upregulated (Up) or downregulated (Down) genes in each region. There is an association between gene expression and chromosomal aberrations for the genes in the regions of frequent gains and losses (P<0.0001; Fisher’s exact test). Figure 1: Chromosomal aberrations regulating expression of genes from frequent chromosomal gain or loss. ( a ) Heat map of the 1,268 genes differentially expressed between cervical tumour and normal tissue samples in the five data sets used for the meta-analysis of gene expression microarray data. red-upregulated, green-downregulated, grey-missing value. *Current study. ( b ) FqG (red) or loss (FqL, green) in the genome detected in the meta-analysis of comparative genomic hybridization studies using cervical cancer samples. ( c ) Distribution of the delta values (FqG—FqL) for the 1,268 genes. Chromosomal regions with delta values >0.32 or <−0.2 were considered to be the regions of frequent gains or losses, respectively. Bar graph shows the number of upregulated (Up) or downregulated (Down) genes in each region. There is an association between gene expression and chromosomal aberrations for the genes in the regions of frequent gains and losses ( P <0.0001; Fisher’s exact test). Full size image As the chromosomal imbalances may cause alterations in gene expression, we questioned whether the identified DEGs were located in the regions of frequent chromosomal gains or losses. To identify regions of chromosomal aberrations in cervical cancer we performed a meta-analysis of published comparative genomic hybridization studies in this cancer ( Supplementary Table S2 ). We used a total of 269 cases from ten studies and determined the frequencies of gains and losses for the whole genome ( Fig. 1b ). Next, we retrieved information on chromosomal aberration frequencies for 1268 DEGs according to their gene locations ( Supplementary Fig. S1a , Supplementary Data 2 ) and calculated the difference between frequency of gain (FqG) and frequency of loss (FqL) for each gene. In order to identify the cutoff values for frequent losses and gains, we plotted the density distribution for these differences ( Supplementary Fig. S1b ) and searched for local minima on both sides of the distribution. The cutoff values were −0.2 and 0.32 of (FqG—FqL) for frequent losses and frequent gains, respectively ( Supplementary Fig. S1b ). The frequent loss regions were located on chromosomes 2 (2q33-q37), 3 (3p12-p26), 4 (4p12-p15.2, 4q13-q35), 11 (11q23-q25) and 13 (13q21) and the frequent gain regions on chromosome 3 (3q13.2-q29) ( Supplementary Fig. S1c ). In the loss regions there were 89 DEGs (66 Down- and 23 Up-genes), and in the gain regions 62 DEGs (53 Up- and 9 Down-genes) ( Fig. 1c ). Thus, we found a strong association between chromosomal gains or losses and upregulation or downregulation of gene expression ( P <0.0001; Fisher’s exact test), indicating that the majority of DEGs located in the regions of frequent chromosomal aberrations are regulated by these aberrations. Gene network reconstruction and identification of subnetworks Although we found that chromosomal aberrations regulated the expression of about 80% of DEGs located within these regions, those genes represented only ~9% of all DEGs. It is known, however, that DEGs are not totally independent from each other but rather represent a regulatory network driven by different factors, with chromosomal aberrations being one of them. Therefore, some DEGs can be indirectly regulated by chromosomal gains or losses, if their expression is regulated by another gene directly affected by a chromosomal aberration. To uncover such regulatory relationships we employed an approach of network reconstruction that we have previously applied to disclose gene–gene interactions in immunodeficiency [10] . We analysed correlations between all gene pairs formed by the DEGs and found 3,161 correlated gene pairs with FDR ≤0.1%. The network was composed of 738 genes with only a few gene pairs not connected to the main network ( Fig. 2 ; P <10 −300 ; Erdős–Rényi model, see Supplementary Methods ). We analysed this network to find subnetworks, which may have specific biological functions. We found three major subnetworks that contained 112 genes (sub-network 1), 54 (sub-network 2) and 19 genes (sub-network 3), respectively ( Fig. 2 ). Using functional enrichment analysis, we identified ‘cell cycle’ (sub-network 1), ‘response to virus’ (sub-network 2, which we name ‘antiviral’ in the manuscript) and ‘epithelial cell differentiation’ (sub-network 3) as the main Gene Ontology terms overrepresented in these subnetworks ( Supplementary Table S3 ). The cell cycle and antiviral subnetworks consisted mostly of upregulated genes and the epithelial cell differentiation subnetwork of downregulated genes. 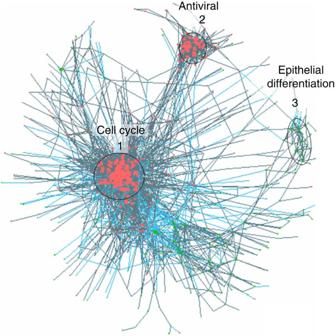Figure 2: Gene regulatory network reconstructed using the DEGs in cervical cancer. Dots are genes (red, upregulated; green, downregulated); lines indicate the presence of correlation between genes. The three identified subnetworks indicated by circles were named after Gene Ontology terms they represent as Cell Cycle, Antiviral (equivalent to GO term ‘response to virus’), and Epithelial differentiation. Figure 2: Gene regulatory network reconstructed using the DEGs in cervical cancer. Dots are genes (red, upregulated; green, downregulated); lines indicate the presence of correlation between genes. The three identified subnetworks indicated by circles were named after Gene Ontology terms they represent as Cell Cycle, Antiviral (equivalent to GO term ‘response to virus’), and Epithelial differentiation. Full size image Hierarchy in the subnetworks To search for key regulators of the process and to test the regulatory relationships among the genes, we needed to establish a hierarchy within the subnetworks. It was previously shown for different cancers that alteration in expression of genes located within chromosomal aberration can be a critical event driving a disease [11] . Furthermore, we based our analyses on a mathematical/statistical concept that correlation is a result of causation unless it is found by chance. The correlations, according to ‘Reichenbach’s common cause principles’ [12] , [13] , should reflect regulatory relationships. Specifically, if there is a correlation between expression of gene X and Y, then there are three possibilities: X regulates Y, Y regulates X or there is Z that regulates both. Thus, for the case when X correlates with Y and there is a known cause for X (that is, chromosomal aberration) the most likely scenario will be that X regulates Y (see Supplementary Fig. S2 ). We used two criteria for ranking genes within subnetworks for their potential to be key regulators: first, frequency of chromosomal aberrations in patient population concordant with a direction of the change in gene expression (that is, gain corresponding to upregulation; loss to downregulation). Second criterion was the number of connections with other genes in the network, as this feature had been shown to be a distinctive characteristic of major regulators [14] . The top-ranked genes were considered as gene-regulators and placed on the top of the hierarchy, followed by the genes directly linked to them (targets) and then by the genes that did not have direct links to the regulators. We could establish these hierarchies for subnetworks 1 ( Fig. 3a ) and 2 ( Fig. 3b ), but not for subnetwork 3 ( Supplementary Fig. S3a ) as there was no gene that met the first criterion of a regulator in this subnetwork. 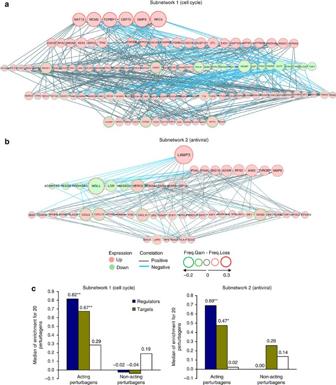Figure 3: Hierarchy in the cell cycle and antiviral subnetworks. (a) Subnetwork 1—Cell Cycle. (b) Subnetwork 2—Antiviral. The subnetworks 1 and 2 have genes located in the regions of frequent DNA gain and were organized hierarchically with the regulator genes on the top and the target genes below them. (c) Testing the hierarchy of the subnetworks by perturbagens analysis using the Connectivity Map (http://www.broadinstitute.org/cmap). Twenty acting and 20 non-acting perturbagens were tested in each group of genes (regulators, targets and other subnetwork), in the subnetwork 1 and subnetwork 2. Enrichment score (or connectivity score) is a measure of how perturbagens influence a gene expression signature where high-positive score means significant induction (designated by **P<0.0001 and *P<0.001; Mann–Whitney test). Figure 3: Hierarchy in the cell cycle and antiviral subnetworks. ( a ) Subnetwork 1—Cell Cycle. ( b ) Subnetwork 2—Antiviral. The subnetworks 1 and 2 have genes located in the regions of frequent DNA gain and were organized hierarchically with the regulator genes on the top and the target genes below them. ( c ) Testing the hierarchy of the subnetworks by perturbagens analysis using the Connectivity Map ( http://www.broadinstitute.org/cmap ). Twenty acting and 20 non-acting perturbagens were tested in each group of genes (regulators, targets and other subnetwork), in the subnetwork 1 and subnetwork 2. Enrichment score (or connectivity score) is a measure of how perturbagens influence a gene expression signature where high-positive score means significant induction (designated by ** P <0.0001 and * P <0.001; Mann–Whitney test). Full size image In order to test the hierarchies of the subnetworks in the experimental settings, we took an advantage of the CMAP database [15] , which contains global gene expression data of in vitro responses to a big variety of perturbations. First, we divided each subnetwork into two groups of genes: the first mainly containing regulators and the second one targets ( Supplementary Fig. S3b,c ). We tested the hypothesis that perturbagens that stimulate regulators should also stimulate targets of the given subnetwork. For each subnetwork we chose 20 perturbagens, which induced regulators (that is, acting perturbagens). Next, we tested if these perturbagens also acted on the target genes. As controls, we also selected perturbagens, which did not act on the regulator genes (non-acting perturbagens). As a specificity control, we tested these perturbagens on the genes from the other subnetwork. For both subnetworks, we observed that perturbagens selected on the basis of their ability to stimulate regulators also stimulated targets of a given subnetwork, but not genes of another subnetwork ( Fig. 3c ). Perturbagens with no effect on regulators did not show any effect on the targets either. Therefore, these results give us experimental support for the two ideas emerging from network analysis: first, no or minimal cross-regulation between genes of different subnetworks; and the second, that genes defined as regulators can drive the expression of target genes from the same subnetwork. It is important, though, to interpret these results in combination with other data because in isolation they do not rule out a possibility that regulators and targets are under common regulatory mechanisms affected by perturbagens. Validation of genomic aberrations and gene expression network Although the meta-analyses of chromosomal aberrations and gene expression network were performed using many independent studies, we wanted to validate these results by analysing another cohort of patients. For this, we used an independent data set containing comparative genomic hybridization data on 97 patients with cervical cancer [16] and obtained gene expression data for 82 of them. First, we checked for the overall concordance of the genomic aberrations of the drivers/regulators genes between this new data set and our meta-analysis. We observed a remarkably strong correlation between the two results ( r =0.8, P <0.0001, Pearson correlation, Fig. 4a ) further supporting the idea that genomic aberrations in those genes are a general feature of invasive cervical cancers. 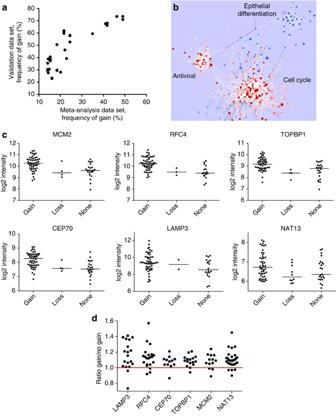Figure 4: Reproducibility of the meta-analysis in a new patient data set. (a) Correlation between FqG in the meta-analysis and in validation data set for the 36 regulator genes from the cell cycle and antiviral subnetworks (r=0.8;P<0.0001; spearman rank correlation). (b) Gene expression data of 82 patients were used to build a network from the genes that comprised the meta-network. Red nodes are upregulated genes, blue nodes are downregulated genes, white and black edges represent positive and negative correlations, respectively. Three subnetworks are indicated. (c) Chromosomal gains increase expression of key driver genes. Expression level of each of the six genes in patients with gains, losses or no change in the corresponding chromosomal region. Each symbol represents an individual tumour.NAT13, LAMP3,P<0.01; others,P<0.001 for comparison of ‘gain’ versus ‘none’. (d) Chromosomal gains in the key driver genes regions regulate expression of their respective target genes. Driver genes are indicated onxaxis. Each dot represents ratio for individual target genes that are calculated by dividing average expression of a target gene in tumors with gains by its expression in tumours with no gains. Figure 4: Reproducibility of the meta-analysis in a new patient data set. ( a ) Correlation between FqG in the meta-analysis and in validation data set for the 36 regulator genes from the cell cycle and antiviral subnetworks ( r =0.8; P <0.0001; spearman rank correlation). ( b ) Gene expression data of 82 patients were used to build a network from the genes that comprised the meta-network. Red nodes are upregulated genes, blue nodes are downregulated genes, white and black edges represent positive and negative correlations, respectively. Three subnetworks are indicated. ( c ) Chromosomal gains increase expression of key driver genes. Expression level of each of the six genes in patients with gains, losses or no change in the corresponding chromosomal region. Each symbol represents an individual tumour. NAT13, LAMP3 , P <0.01; others, P <0.001 for comparison of ‘gain’ versus ‘none’. ( d ) Chromosomal gains in the key driver genes regions regulate expression of their respective target genes. Driver genes are indicated on x axis. Each dot represents ratio for individual target genes that are calculated by dividing average expression of a target gene in tumors with gains by its expression in tumours with no gains. Full size image Next, we wanted to ensure the reproducibility of the gene expression meta-network. Using gene expression data of 82 tumours, we analysed connections of the meta-network in the new data and found that ~96% of the significant correlations (FDR <10%) had the same directions as in the original network. Next we analysed the substructure of this network and found three major subnetworks, which corresponded to those previously revealed in the original meta-network ( Fig. 4b ). Remarkably, each of the three subnetworks contained about 90% of genes out of the original subnetworks and all but one of the identified major key regulators were within the subnetworks. After a detailed inspection, we found that the missing major regulator gene ( GMPS ) actually does not have a probe on the Illumina platform that we have used for this new experiment. Overall, these results show that the meta-network we have reconstructed is highly reproducible in a new set of patients, demonstrating the robustness of our approach to meta-network reconstruction. As the validation patient data set had both genomic aberrations data and gene expression data, we could directly ask whether the chromosomal gains in the key driver genes influence their expression. We found (as was predicted by our previous analysis, Fig. 1c ) that expression of the key drivers was higher in tumours that had chromosomal amplifications in regions where these genes were located than in tumours with no aberrations or with losses in these regions ( Fig. 4c ). Next we asked whether the genes we predicted to be the targets of the key drivers have different expression depending whether the drivers have chromosomal gains or not. We tested this question by comparing the expression signature of target genes directly connected in the meta-network to the six driver genes between tumours with and without gains for the driver genes. To avoid biases, we only tested those target genes that were not located on the same chromosome with their corresponding driver. We observed that the signatures of target genes respective to each key driver had higher expression in tumours with gains than in tumours with no gains (loss and no aberration), suggesting that majority of the targets are to be regulated by their respective driver genes ( Fig. 4d ). These new results give an independent experimental support for our claim that the key driver genes we identified may drive the expression of the genes connected to them in the network. Frequent aberrations contain cell cycle and antiviral drivers Although both the cell cycle and antiviral subnetworks were upregulated in tumours, we observed only a few correlations between gene expression of these two subnetworks. As regulator/driver genes for both of these subnetworks were located in the regions of frequent chromosomal gains, we hypothesized that there might be relationships between the two subnetworks at the genomic level. In this analysis, we could only include the 117 patients from the meta-analysis whose individual data on genomic aberrations were available, as wells as data from 97 patients of the validation data set [16] . We asked if aberrations in the regions with the drivers of two functional classes (antiviral and cell cycle) appear in different samples reflecting the heterogeneity of cervical cancer or if these aberrations are present in the same tumours. In the meta-analysis and the validation data set, we found a much higher frequency of copresence of the aberrations in regions that contained cell cycle and antiviral drivers in the same samples than might be expected by chance (meta-analysis data set: P <0.0001, validation data set: P <0.002; χ 2 -test, Fig. 5a ). 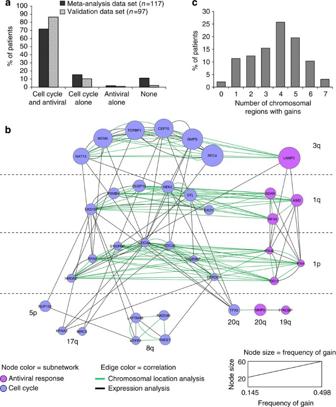Figure 5: Drivers of cell cycle and antiviral subnetworks are located in the same regions of frequent gains. (a) Frequency of patients with chromosomal gains containing the driver genes from the cell cycle and Antiviral subnetworks together and separately in the patients from meta-analysis and from validation data set (P<0.0001,P<0.002,χ2-test respectively). (b) An integrative network reconstructed with data on chromosomal aberrations and gene expression correlation using the driver genes of cell cycle and antiviral subnetworks. All correlations in this network were positive. (c) Distribution of number of frequent chromosomal aberrations (gains) present in the same tumour. The regions used for this analysis were those containing regulator genes (1q, 1p, 3q, 5p, 8q, 17q, 19q, 20q). Forbandc,n=97 patients from the validation data set. Figure 5: Drivers of cell cycle and antiviral subnetworks are located in the same regions of frequent gains. ( a ) Frequency of patients with chromosomal gains containing the driver genes from the cell cycle and Antiviral subnetworks together and separately in the patients from meta-analysis and from validation data set ( P <0.0001, P <0.002, χ 2 -test respectively). ( b ) An integrative network reconstructed with data on chromosomal aberrations and gene expression correlation using the driver genes of cell cycle and antiviral subnetworks. All correlations in this network were positive. ( c ) Distribution of number of frequent chromosomal aberrations (gains) present in the same tumour. The regions used for this analysis were those containing regulator genes (1q, 1p, 3q, 5p, 8q, 17q, 19q, 20q). For b and c , n =97 patients from the validation data set. Full size image In order to understand the nature of this copresence we reconstructed a chromosomal aberration network between gene-regulators of the cell cycle and antiviral subnetworks. As only the validation data set contained quantitative values of the level of chromosomal amplification for each gene in each patient, we used this data set to analyse correlations between these values and to reconstruct a network ( Fig. 5b ). As expected, genes located in a physical (that is, genomic) proximity to one another showed high correlations at the level of genomic aberrations (green edges, Fig. 5b ) despite their affiliations with different gene expression subnetworks (cell cycle and antiviral). Note that genes for several other processes are located in the same chromosomal gains as cell cycle and antiviral gene drivers. Many of those genes were also among differentially expressed but they were not classified as drivers in the analysis. For example, in the frequently gained region 3q13.2 to 3q27.3, there were 46 overexpressed genes but only seven were identified as regulators. Thus it’s only a minority of the genes located within frequent chromosomal aberrations that are identified as regulators by our analysis, but all of those represented either cell cycle or antiviral genes. We next asked if each tumour contained aberrations from only one chromosomal region. This was not the case. The majority of tumours contained gains in four or more chromosomal loci with a total of 58 unique combinations across 97 tumours ( Fig. 5c ; Supplementary Fig. S4 ). Differently from the link between cell cycle and antiviral drivers, we did not find any particularly preferred combination pair. For example, two most frequent aberrations in 3q and 1q appear in 76% and 64% of tumours, respectively. The proportion of tumours where these two aberrations co-occur is ~50%, which is almost the same as would be expected by chance (48%). The analysis of more complex combinations (three to seven aberrations) was precluded by the available sample size. Thus, altogether these results suggested that the combinations of frequent chromosomal aberrations that contain cell cycle and antiviral drivers seem to be necessary for the development of invasive carcinoma indicating potential synergy between the two biological processes. LAMP3 as a regulator of antiviral genes in cervical cancer The increased activity of the cell cycle genes and decreased epithelial differentiation are well known attributes of different malignancies, including cervical cancer [17] . The finding of increased expression of genes related to the antiviral response was surprising, because persistent high-risk HPV infection is highly associated with malignancy [1] . Among these genes there were innate immune sensors of viruses ( ADAR, AIM2 ), molecules involved in antigen presentation ( HLA, TAP, RFX5 ), transcription regulators ( IRF1, IRF7, IRF9 , and STAT1 ) and other genes of innate immunity (such as HERC5, MX1, OAS2, ISG15 , and RSAD2 (viperin)) directly involved in the elimination of viruses [18] , [19] . In order to test whether the antiviral subnetwork genes would be active in other infections, we compared expression of this signature between cervical cancer and several viral and bacterial infections. The great majority of the genes of the antiviral subnetwork were concordantly regulated in cervical cancer and in influenza virus, rhinovirus and respiratory sincitial virus infections, whereas there was no similarity to bacterial infections ( Supplementary Fig. S5 ), indicating that cervical cancer has gene expression properties of activated antiviral response represented by genes of the corresponding subnetwork. In order to test if genes we have predicted as antiviral from ex vivo tumour data are actually regulated in the context of a well-defined experimental HPV infection, we took advantage of the gene expression data obtained in the in vitro W12 system of cervical carcinogenesis [8] . In this model, the authors demonstrated that outgrowth of HPV-integrated cells was associated with the loss of episomal HPV and simultaneous activation of antiviral response. Therefore, we tested if the genes from the antiviral subnetwork we found in patients were associated with the loss of episomal virus in this in vitro system. From the 54 genes of antiviral subnetwork, 36 were detected in the vitro model, and of those, 18 were significantly regulated (FDR<10%), with 16 out of 18 genes having higher expression during episomal HPV elimination in vitro ( Fig. 6a ). Out of 18 genes that did not pass the threshold, 11 also had higher expression at the stage of episomal E2 drop. This result supports the idea that activation of antiviral genes in vivo might be involved in the elimination of episomal virus in tumours. Further, analysing effect of interferon treatment we found that tumour-derived antiviral signature contained pathways dependent on both types of interferon ( Supplementary Fig. S6 ). 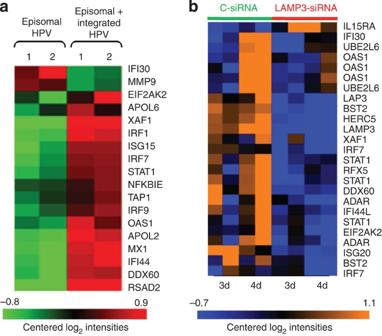Figure 6: Antiviral subnetwork genes are regulated by LAMP3. (a) Expression of genes from the antiviral subnetwork in anin vitroculture W12 before and during elimination of episomal HPV in the presence of integrated HPV in the study of Pettet al. (data retrieved from GSE4289). (b) Knockdown of LAMP3 by siRNA leads to downregulation of many antiviral IFN-dependent genes. HeLa cells were pretreated with control or LAMP3 siRNA overnight, then 1 ng ml−1IFN-alpha was added for 3 or 4 days and gene expression was assessed. Log intensity values are represented by colours: orange—high expression, blue—low expression. Figure 6: Antiviral subnetwork genes are regulated by LAMP3. ( a ) Expression of genes from the antiviral subnetwork in an in vitro culture W12 before and during elimination of episomal HPV in the presence of integrated HPV in the study of Pett et al . (data retrieved from GSE4289). ( b ) Knockdown of LAMP3 by siRNA leads to downregulation of many antiviral IFN-dependent genes. HeLa cells were pretreated with control or LAMP3 siRNA overnight, then 1 ng ml −1 IFN-alpha was added for 3 or 4 days and gene expression was assessed. Log intensity values are represented by colours: orange—high expression, blue—low expression. Full size image We demonstrated that LAMP3 was one of the major regulators of antiviral subnetwork with chromosomal amplifications of its genomic region occurring in >50% of patients. Although this gene is known to be regulated by interferon [20] and might be involved in antigen presentation [21] , its precise role in immune response is uncertain. Therefore, we decided to further test the role of LAMP3 as a regulator of antiviral genes. We compared the expression signature of the genes from the antiviral subnetwork between LAMP3 short interfering RNA (siRNA) and control siRNA-treated HeLa cells after interferon stimulation. All 17 genes but one (IL15RA) that showed significant difference (FDR<10%) in gene expression between cells treated with control- and LAMP3-siRNA were regulated as predicted by our meta-analysis, that is had lower expression in cells where LAMP3 was knocked down ( Fig. 6b ). Several well-known interferon (IFN)-dependent antiviral genes such as STAT1, IRF7, HERC5, ISG20 and OAS1 were affected by LAMP3 downregulation. Thus, taking together the knockdown and chromosomal amplification results, we conclude that LAMP3 has a key regulatory role in the activation of interferon-dependent antiviral genes in cervical cancer. As only a small percentage of women harbouring the virus develop the cancer [22] , HPV infection alone appears to be insufficient for the progression of cervical cancer [23] . Thus, the interaction between the infected cells, immune system and virus seems to be involved in the malignant progression of cervical cancer. Aiming to understand this complex process, we started by integrating global transcriptional profiling and genomic data and found that only small proportion (~9%) of DEGs can be directly regulated by frequent chromosomal aberrations. This result led us to hypothesize that the genes regulated by chromosomal aberrations might themselves regulate other genes. To substantiate this claim, we reconstructed a coexpression gene network of cervical cancer. There were multiple pieces of evidence indicating that this coexpression network reflects causative relationships between genes. First, we found that in vitro perturbation of major regulators of each individual subnetwork, located within chromosomal amplifications, resulted in a similar effect on target genes of the same sub-network, but did not affect unrelated genes ( Fig. 3c ). Second, using independent cohort of patients in whom we could obtain gene expression and genomic aberrations data we demonstrated that genes predicted to be targets of key drivers had higher expression in tumours with genomic gains than in tumours without gains for respective drivers ( Fig. 4d ). The last but not the least, we showed that in vitro knockdown of LAMP3 leads to downregulation of many antiviral genes predicted to be stimulated by this molecule by our analysis. Altogether these findings strongly support our model that majority of transcriptional events in cervical cancer are directly and indirectly driven by chromosomal aberrations. The identification of two subnetworks, cell cycle and epithelial cell differentiation, was not surprising, as both were extensively studied in cervical cancer [17] . From the cell cycle subnetwork, six genes ( CEP70, GMPS, MCM2, NAT13, RFC4 and TOPBP1 ) located in regions of frequent chromosomal aberrations were identified as the main drivers in this subnetwork. All these genes are located on chromosome 3q, where a frequent DNA gain occurs. This amplification has been previously described in cervical cancer [24] . Although some of these genes have been also demonstrated as regulated by chromosomal gains, our study is the first to point to their key role in driving cell cycle transcriptional programme in cervical cancer. The increased expression of antiviral genes was surprising, because one could expect a reduction in the antiviral response to occur during persistent HPV infection as E6/E7 proteins were shown to inhibit interferon related responses [25] . The natural history of infection, however, shows that in most cases antiviral response prevails over the inhibitory activity of HPV as ~90% of women eliminate the virus. Also, Pett et al . [8] made an interesting observation in an in vitro system that activation of antiviral immune response genes was associated with the loss of episomal HPV16, overexpression of E6/E7 oncogenes and outgrowth of cervical keratinocytes containing integrated HPV. These results led them to propose a model of cervical carcinogenesis where elimination of episomal virus, by activated immune response, is a critical step in tumour progression because it removes the inhibitory component of the episomal virus (E2) and releases oncogenes expression [2] . Although the new model [8] insightfully proposed the antiviral response as a critical step in tumour progression, the trigger of this gene activation, remained a mystery. Our results provide the first in vivo evidence that chromosomal amplifications in the antiviral genes selected during cancer development trigger and sustain their activation in the tumour possibly providing additional help for the host immune system, which was unable to eliminate the virus alone. It is remarkable that regions of frequent chromosomal gains simultaneously contained drivers not only of antiviral but also of cell cycle genes in the majority of patients ( Fig. 5 ). This result indicates that both processes might be necessary for tumour survival and, as might be expected, it would be cost-effective to select one aberration that simultaneously affects both functions (that is, killing two birds with one stone). Activation of the two processes may have synergistic effect on the tumour progression, because while antiviral response ultimately would lead to the block of cell cycle repressors (p53 and retinoblastoma) by permitting overexpression of E6/E7, the second group of drivers directly promotes cell cycle ( Fig. 7 ). Although this is the most plausible model, other interpretations may exist such as that stimulation of immune response by ‘antiviral’ drivers might be tumour-promoting independently on the episomal HPV decline. 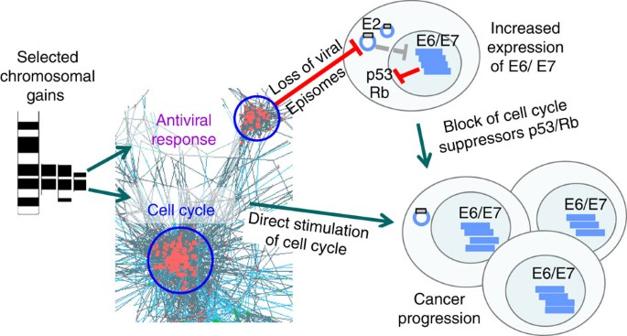Figure 7: A revised model of cervical carcinogenesis. Persistent high-risk HPV infection may result in the integration of virus into host genome leading to the increased genomic instability and aberrations, however, the expression of E6/E7 oncogenes is still under control of E2 if the episomal virus is around. If the chromosomal aberrations (gains) occur in the regions containing antiviral genes, they will induce the elimination of inhibitory episomal E28, release of E6/E7 that will block suppressors of cell cycle (p53, retinoblastoma). The same chromosomal gains contain drivers of cell cycle that directly induce cell proliferation. The two processes act synergistically allowing the dysplastic cell to become a malignant tumour. Figure 7: A revised model of cervical carcinogenesis. Persistent high-risk HPV infection may result in the integration of virus into host genome leading to the increased genomic instability and aberrations, however, the expression of E6/E7 oncogenes is still under control of E2 if the episomal virus is around. If the chromosomal aberrations (gains) occur in the regions containing antiviral genes, they will induce the elimination of inhibitory episomal E2 [8] , release of E6/E7 that will block suppressors of cell cycle (p53, retinoblastoma). The same chromosomal gains contain drivers of cell cycle that directly induce cell proliferation. The two processes act synergistically allowing the dysplastic cell to become a malignant tumour. Full size image One of the major drivers of the antiviral sub-network, LAMP3 , was the only driver from this subnetwork located in the same gain region (3q) as the cell cycle drivers. An overexpression of this gene has been associated with the enhanced metastatic potential and poor prognosis in cervical cancer [26] . It was not clear, however, which cellular process is affected and leads to cancer progression as a result of LAMP3 elevation. Our results suggest that this gene is one of the major drivers of immune/antiviral genes activated in the process of cervical oncogenesis, a result that can hardly be obtained without the comprehensive reconstruction and analysis of a genomic/transcriptomic network. Although LAMP3 had not been shown before as a regulator of immunity, its increased expression was associated with better response to antiviral treatment in patients with Hepatitis C ( [27] ). Thus, our results in tumours ( Fig. 4d ) and knockdown of LAMP3 by siRNA in cell line ( Fig. 6b ) is the first direct demonstration that LAMP3 drives the IFN-dependent gene expression signature, which is highly enriched for antiviral genes such as STAT1, IRF7, HERC5, ISG20 , OAS1 among others. Taken together with the findings that LAMP3 is involved in the cancer metastatic process [26] , these results suggest that LAMP3 may have a dual role in cervical cancer promoting expression of antiviral genes and possibly contributing to elimination of episomic HPV and increasing the migratory capacity of tumour cells. Other regulators of the antiviral subnetwork were located outside of 3q in chromosomes 1 and 20 but it was recently shown that those regions also have characteristic aberrations in advanced intraepithelial lesions with a high short-term risk for progression [28] . Furthermore, in vitro modulation of expression of RFX5 ( [29] ) and AIM2 ( [30] ), located on 1q, leads to the expected changes in expression of predicted targets ( Supplementary Fig. S7 ). Interestingly, of the nine genes from the antiviral subnetwork regulated by chromosomal aberrations and considered to be regulator genes, eight are located on these regions (3q, 1q, 1p, 20q). Herein we show that antiviral genes we found overexpressed in cervical cancer are active in several viral but not bacterial infections ( Supplementary Fig. S5 ), suggesting that host uses common mechanism for elimination of different viruses including HPV. These genes contain a mixed pattern of IFN type I and type II pathways, while the in vitro results of Pett et al . [8] indicated an involvement of only type I interferon. This partial discrepancy can probably be explained by the mixture of different cell types, including immune cells, that generates antiviral signature in vivo . This hypothesis is supported by the fact that expression of some genes from antiviral subnetwork is known to be limited to immune cells (for example, CD163, FCGR1B and granzyme B; Supplementary Fig. S8 ). In addition, it agrees with the data showing that high expression of granzyme B is associated with poor outcome of cervical cancer patients [31] . In contrast to the cell cycle and antiviral subnetworks, we did not find any evidence that protein coding genes located within chromosomal aberrations can be regulators of the epithelial differentiation subnetwork. Our bioinformatics analysis ( Supplementary Methods ; Supplementary Fig. S9 ), however, indicated that the genes from this subnetwork might be downregulated by mir-15b and mir-16-2 that are located within amplification in 3q region and had been already shown overexpressed in cervical cancer [32] , [33] , [34] . A recent paper using a similar strategy has discovered major drivers of a melanoma [11] . Thus, the successful application of this approach in such different malignancies as cervical cancer and melanoma suggests its potential usefulness for the analysis of almost any tumour, as genomic aberrations are generic features of malignancies. Akavia et al . [11] demonstrated that their algorithm discovers critical drivers of carcinogenesis in ‘any tumour cohort containing matched data for copy number aberrations and gene expression’. The critical advantage of our approach is that we have revealed key drivers of the process using non-matched genomic and transcriptomic data sets with the only connection between those being the fact that all data were collected from patients with cervical cancer. In summary, by reconstructing and analysing a gene regulatory network of cervical cancer, we infer a model of carcinogenesis in which genomic aberrations that promote cell cycle progression and elimination of episomal HPV are the major drivers of the process and orchestrate the growth advantage of the tumour cells carrying them ( Fig. 7 ). In addition to the novel analytical approach and surprising biological insight, our study has potentially important implications for future clinical practice. For example, current World Health Organization guidelines on HPV vaccination do not contain any specific recommendations in regard to HPV status of the vaccine recipient [35] . Also, anti-HPV therapy with immune-modulators inducing interferon pathways has been proposed to treat HPV-infected women [36] . Our results, however, suggest that antiviral therapy or anti-HPV therapeutic vaccination might be dangerous for women whose lesions already present signs of HPV integration. Furthermore, we compiled a comprehensive list of genomic and transcriptomic markers that if detected in preinvasive cancer lesions might be indicative of poor prognosis. Meta-analysis of gene expression data We searched PubMed at the NCBI database ( http://www.ncbi.nlm.nih.gov/pubmed/ ) for studies of microarray in cervical cancer (published until 03/2009) and selected four studies [37] , [38] , [39] , [40] that: (i) had publicly available microarray data, (ii) used tumour and normal clinical samples, (iii) used oligonucleotide arrays and (iv) had sample size in each class ⩾ 5 ( Supplementary Table S1 ). The data were analysed using BRB Array-Tools v3.6.0 beta 3 developed by Drs Richard Simon and Amy Peng Lam ( http://linus.nci.nih.gov/BRB-ArrayTools.html ) using the original normalization used in three studies [37] , [38] , [40] and median normalization over entire the array for the fourth study [39] . For all studies, we only considered genes found in at least 70% of arrays. Besides publicly available data used in this study, we analysed gene expression in samples collected from two unrelated cohorts of patients, first one became a part of meta-analysis and the second was used for validation. The first data set consisted of cervical cancer biopsies ( n =40) and normal adjacent tissue samples ( n =20) (Gene Expression Omnibus accession code GSE26342 ). The second data set consisted of cervical cancer samples from 82 patients (GSE27469). See details of both cohorts in Supplementary Methods . DEGs between tumour and normal samples were identified for each of the five studies using random-variance t -test and then combined in a meta-analysis using Fisher’s inverse χ 2 -method [41] as described in Supplementary Methods . Meta-analysis of comparative genomic hybridization data We selected ten publications, which studied tumour clinical samples and provided either individual comparative genomic hybridization data for their samples or graphical diagrams [42] , [43] , [44] , [45] , [46] , [47] , [48] , [49] , [50] , [51] . A total of 269 cervical cancer cases were identified from the ten studies ( Supplementary Table S2 ). From each study, we extracted the number of cases with chromosomal aberrations (gain and loss) in each chromosomal band to calculate the FqG, FqL and the delta between them (FqG–FqL). We used the standard ISCN 1995 (an International System for human Cytogenetic Nomenclature 1995) resolution at the 400-band level [52] . Chromosomal gains and losses in each study were defined according to the thresholds reported in the original papers. Integration of gene expression and chromosomal aberrations The chromosomal locations of the 1,268 DEGs identified in the gene expression meta-analysis were determined using the NCBI database. When we did not find the location, we searched the Ensembl database. Based on the chromosomal location, the values of the frequencies (FqG, FqL and delta FqG-FqL) were identified for each gene. We used the delta values of all genes to construct a histogram that displayed their distribution ( Supplementary Fig. S1b ). Using this distribution, we determined the delta values, which were considered to be the cutoffs that identify regions with frequent gain or loss. These were the values of local minima on both sides of the distribution. We applied the Fisher’s exact test to test if the altered expression of genes in these regions was significantly associated with chromosomal aberrations. A P -value <0.05 was considered significant. Reconstruction of the gene expression meta-network Using gene expression data from tumours in five data sets, we calculated correlations between gene pairs [53] and reconstructed networks by performing meta-analysis of correlations using similar approach employed for gene expression. The networks were visualized in the Cytoscape Software 2.6.3 ( [54] ). To identify subnetworks of correlated genes, we used MCODE v1.2 (Molecular Complex Detection) plug-in for Cytoscape [55] . To establish a hierarchy within the subnetworks, we organized the genes as follows: first line, genes located in regions of frequent chromosomal aberrations and with 12 or more links (see Supplementary Methods for estimation of links number); second line, genes located in regions with less frequent chromosomal aberrations (delta values between −0.2 and −0.1 and between 0.1 and 0.32); third line, genes directly connected with genes from the first line; fourth line, genes connected with genes from the second line; last line, the rest of the genes. Genes in lines 3 and further did not have chromosomal aberrations (delta −0.1 to 0.1). See details in Supplementary Methods . Perturbagens analysis We used the Connectivity Map 02 (CMAP) [15] to perform the perturbagen analysis. The genes of each subnetwork were divided into two groups: regulators and targets ( Supplementary Fig. S3 ). The regulator genes were used to select the perturbagens and the target genes to test them. As controls, we used genes from another subnetwork and we also analysed perturbagens, which did not act on the regulator genes. In total, we selected 20 perturbagens that acted on the regulator genes and 20 that did not do so. See details in Supplementary Methods . Chromosomal aberrations network We used data from our meta-analysis with the available individual patient results on genomic aberrations ( n =117) and results from another independent data set [16] ; ArrayExpress accession no. E-TABM-398 for reconstruction of a chromosomal aberrations network. We reconstructed the genomic aberrations network using the same approach employed for reconstruction of gene expression network (details in Supplementary Methods ). LAMP3 knockdown experiment HeLa cells obtained directly from American Type Culture Collection were transfected with LAMP3-specific siRNA or control siRNA (ON-TARGETplus SMARTpool), then stimulated with interferon and gene tested for genes expression as described in Supplementary Methods . Accession codes: Gene expression data have been deposited in the Gene Expression Omnibus under accession codes GSE26342 (40 cervical cancer biopsies and 20 normal adjacent tissue samples), and GSE27469 (validation dataset of cervical cancer samples from 82 patients). How to cite this article: Mine, K. L. et al . Gene network reconstruction reveals cell cycle and antiviral genes as major drivers of cervical cancer. Nat. Commun. 4:1806 doi: 10.1038/ncomms2693 (2013).